Synergistic toughening of composite fibres by self-alignment of reduced graphene oxide and carbon nanotubes The extraordinary properties of graphene and carbon nanotubes motivate the development of methods for their use in producing continuous, strong, tough fibres. Previous work has shown that the toughness of the carbon nanotube-reinforced polymer fibres exceeds that of previously known materials. Here we show that further increased toughness results from combining carbon nanotubes and reduced graphene oxide flakes in solution-spun polymer fibres. The gravimetric toughness approaches 1,000 J g −1 , far exceeding spider dragline silk (165 J g −1 ) and Kevlar (78 J g −1 ). This toughness enhancement is consistent with the observed formation of an interconnected network of partially aligned reduced graphene oxide flakes and carbon nanotubes during solution spinning, which act to deflect cracks and allow energy-consuming polymer deformation. Toughness is sensitive to the volume ratio of the reduced graphene oxide flakes to the carbon nanotubes in the spinning solution and the degree of graphene oxidation. The hybrid fibres were sewable and weavable, and could be shaped into high-modulus helical springs. Strong, tough, lightweight polymer fibres are of great interest for various applications, ranging from composites for vehicles to bulletproof vests. Incorporation of electrically conductive additives, such as carbon nanotubes (CNTs), into these fibres can both improve mechanical properties and enable the multi-functionality needed for electrical energy storage [1] , sensing [2] , [3] and actuation [4] . Many of the possible applications would greatly benefit from increased fibre toughness, which is the ability to absorb mechanical energy before rupture. Fibre toughness is dramatically affected by microstructure, and microstructure design is an important area of textile and materials research [5] . Very high toughness (up to 870 J g −1 ) has been reported for composite CNT/poly(vinyl alcohol) (PVA) fibres produced by wet spinning and subsequent mechanical draw of the spun fibres [1] , [6] . Fibre toughness strongly depended upon the CNT alignment in the fibre axis direction and the extent of polymer chain alignment [6] , [7] . In these previous studies, fibre microstructure was modified by hot and cold drawing of the fibre after spinning, with an intermediate degree of drawing producing the highest toughness [6] , [8] . Methods for preparing tough fibres without the need for a complex drawing process are preferred, both economically and because of difficulties in process control [9] , [10] . Recent studies suggest that the incorporation of chemically reduced graphene oxide flakes (RGOFs) into a polymer matrix can also lead to strong, tough composites [11] , [12] , although providing the additional advantage of reduced cost compared with CNTs [11] . A particularly relevant recent example is the demonstration of tough PVA fibres reinforced with RGOFs, with or without CNTs [13] . The highest toughness estimated from the area under the stress–strain curve was ~310 J g −1 (based on an estimated density of 1.6 g cm −3 ). It was shown that the substitution of RGOFs by CNTs decreased toughness and elongation at break. Also, the exclusive use of GOFs always gave very brittle fibres with an estimated toughness of less than 6 J g −1 . The toughness of the RGOF/PVA fibres was attributed to high elongations resulting from the slippage of partially re-stacked layers of RGOFs, which could not occur in the GOF composites because of the greater extent of hydrogen bonding between the layers [13] . Here we report the formation of super-tough nanostructured fibres by solution spinning of the RGOFs and carbon single-walled nanotubes (SWNTs) into an aqueous PVA solution and demonstrate a strong synergistic effect through hybridization of SWNT and RGOF. We show that a network of the RGOF/SWNT nanoparticles spontaneously forms in fibres during wet spinning when the solution composition and particle dispersion are optimized. Consequently, super-tough fibres were formed without the need for a subsequent drawing process for the as-spun gel state. This fact is explained by strong interactions between the two types of carbon nanoparticles, which provide their mutual self-alignment during solution spinning, thereby creating the fibre microstructure believed to be responsible for dramatically enhanced toughness. 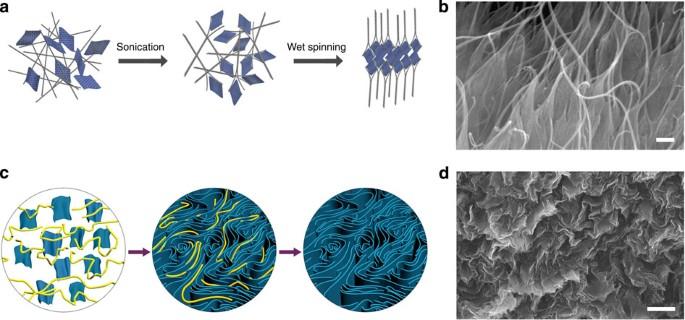Figure 1: Preparation and structure of polymer composite fibres. (a) Schematic diagram showing the formation of the oriented interconnected network of RGOFs (curved rectangles) and SWNT bundles (grey lines) as a result of sonication and subsequent wet spinning. (b) SEM image of the cross-sectional area of a RGOF/SWNT/PVA fibre (1:1 weight ratio of RGOF to SWNT), which clearly shows the co-assembly of RGOFs and SWNTs. Scale bar equals 100 μnm. (c) Schematic illustration of structural evolution between coagulation-spun RGOF gel (left), polymer composite (middle) and polymer-free fibres (right). Yellow lines and blue curved rectangles represent PVA chains and RGOFs, respectively. (d) SEM image of the cross-sectional area of a polymer-free RGOF fibre, which clearly shows the wrinkled RGOFs. Scale bar equals 500 nm. Preparation of graphene-based composite fibres The process for fabricating hybrid fibres based on RGOFs and SWNTs is shown in Figure 1a . Uniform dispersions of various relative amounts of RGOFs and SWNTs in aqueous solutions of sodium dodecyl benzene sulfonate (SDBS) were prepared as described in the 'Methods' section. The aqueous spinning solution, with about pH 7, typically contained 1 wt.% of SDBS and 0.3 wt.% of carbon nanoparticles. Like previously done for SWNTs [8] , [14] , dispersions were then injected into the flow stream of an aqueous solution of 5 wt.% PVA (146,000–186,000 g mol −1 ; hydrolysis, ~99%) dissolved in de-ionised (DI) water, which resulted in coagulation and formation of RGOF/SWNT/PVA-hybrid fibres. After washing in DI water, drying and subsequent methanol treatment to increase PVA crystallinity, we obtained mechanically robust hybrid fibres consisting of RGOF/SWNT nanoparticles imbedded in a PVA matrix ( Fig. 1b ). In all cases, the weight fraction of nanocarbon in the PVA was ~30%. The ratio of RGOF to SWNT in the prepared fibres could be easily controlled by adjusting the ratio of nanoparticles used for the spinning solution. It was also possible to obtain PVA-free fibres by heating the RGOF/PVA fibres in a vacuum at 600 °C for 1 h or by soaking the RGOF/PVA fibres in 37% hydrochloric acid at room temperature for several hours. Figure 1c schematically illustrates the transformation of as-spun gel fibres into solid RGOF/PVA fibres and then polymer-free fibres of wrinkled RGOFs. The polymer-free fibres were mechanically stable, indicating the formation of an interconnected network of RGOFs ( Fig. 1d ). Alternatively, polymer-free fibres could also be produced directly by injecting RGOF/SWNT dispersions into a 37% hydrochloric acid that worked as flocculating agent [15] . Figure 1: Preparation and structure of polymer composite fibres. ( a ) Schematic diagram showing the formation of the oriented interconnected network of RGOFs (curved rectangles) and SWNT bundles (grey lines) as a result of sonication and subsequent wet spinning. ( b ) SEM image of the cross-sectional area of a RGOF/SWNT/PVA fibre (1:1 weight ratio of RGOF to SWNT), which clearly shows the co-assembly of RGOFs and SWNTs. Scale bar equals 100 μnm. ( c ) Schematic illustration of structural evolution between coagulation-spun RGOF gel (left), polymer composite (middle) and polymer-free fibres (right). Yellow lines and blue curved rectangles represent PVA chains and RGOFs, respectively. ( d ) SEM image of the cross-sectional area of a polymer-free RGOF fibre, which clearly shows the wrinkled RGOFs. Scale bar equals 500 nm. 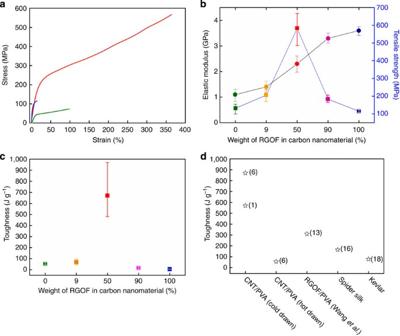Figure 2: Mechanical properties of polymer composite fibres. (a) Stress–strain curves of hybrid (1:1 weight fraction of RGOF to SWNT, red line), SWNT/PVA (green line) and RGOF/PVA (blue line) composite fibres. (b,c) Elastic modulus (circles), tensile strength (squares) (b) and toughness (c) values of fibres with different weight percents of RGOF in total carbon nanomaterials. (d) Comparison of toughnesses of prior-art materials1,6,13,16,18. Error bars inb,crepresent the minimum and maximum values obtained from five independent experiments. Full size image Mechanical properties of graphene-based composite fibres Figure 2a illustrates the striking synergy developed by combining RGOF and SWNT as co-reinforcing materials in our PVA fibres. Using the same processing conditions and precursor carbons (and the absence of either gel-state or solid-state predraw), the strength and elongation at break of the hybrid RGOF/SWNT/PVA fibres were at least three or four times higher than for our SWNT/PVA and RGOF/PVA fibres, respectively ( Fig. 2a,b ). The area under the stress–strain curve in Figure 2a provides the volumetric toughness, which for the 1:1 hybrid RGOF/SWNT/PVA fibres was in the range of 1,015–2,060 MJ m −3 , with an average of 1,380 MJ m −3 . The equivalent mass-normalized toughness is in the range of 480–970 J g −1 ( Fig. 2c ), with the best exceeding the highest values previously reported by Miaudet et al . [6] (870 J g −1 ) and Dalton et al . [1] (570 J g −1 ), which exclusively use SWNTs. These latter values were obtained from solution-spun CNT/PVA fibres that were subsequently stretched in the gel state and then cold-drawn in the dried state by over 100%. The toughness of all of the super-tough fibres far exceed the toughness of other well-known tough fibres such as spider silk (165 J g −1 ) [16] and Kevlar (36–78 J g −1 ) [17] , [18] , and the toughness estimated for the RGOF/SWNT/PVA fibres reported by Wang et al . [13] ( Fig. 2d ). A comparison of the mechanical properties of various graphene-based composite materials is given in Supplementary Figure S1 . Figure 2: Mechanical properties of polymer composite fibres. ( a ) Stress–strain curves of hybrid (1:1 weight fraction of RGOF to SWNT, red line), SWNT/PVA (green line) and RGOF/PVA (blue line) composite fibres. ( b , c ) Elastic modulus (circles), tensile strength (squares) ( b ) and toughness ( c ) values of fibres with different weight percents of RGOF in total carbon nanomaterials. ( d ) Comparison of toughnesses of prior-art materials [1] , [6] , [13] , [16] , [18] . Error bars in b , c represent the minimum and maximum values obtained from five independent experiments. Full size image The synergistic toughening was found to be very sensitive to the ratio of RGOF to SWNTs used in the PVA fibres. The tensile strength and toughness of these composites at first increased and then decreased as the ratio of RGOF to SWNT increased ( Fig. 2b,c ). In contrast, the elastic moduli increased monotonically with the increasing proportion of RGOF incorporated into the fibres ( Fig. 2b ). As the mass fraction of carbon nanoparticles was approximately the same in all fibres, the increasing modulus with higher RGOF content shows that the RGOFs more effectively reinforce the PVA than the SWNTs. The high toughness of the hybrid fibres is also suggested by microscopic features observed using the scanning electron microscopy (SEM; Fig. 3 ). Before stretching, the hybrid fibres show corrugations running along the long axis of the fibre that result from the shrinkage that occurs during coagulation of the precursor as-spun gel fibre ( Fig. 3a ). After stretching to high strains, the fibres show smaller lateral surface corrugation ( Fig. 3b ). It is interesting to note that highly drawn hybrid fibres have periodic wrinkles on their surfaces that are reminiscent of the slip bands sometimes observed on the surface of plastically deformed metals [19] . 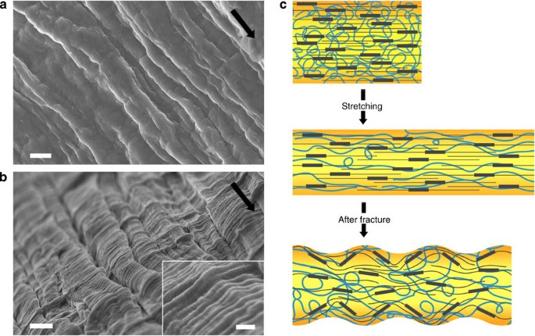Figure 3: Structural changes of hybrid fibres during tensile tests. (a,b) SEM images showing the surfaces of hybrid fibres before stretching (a) and after fracture (b). The arrows of (a) and (b) indicate the fibre axis. Scale bar equals 1 μm, and the inset scale bar in (b) equals 200 nm. (c) Schematic illustrations showing structural changes of hybrid fibres generated during tensile tests. Black rectangles, black lines and blue curved lines are RGOFs, SWNTs and PVA chains, respectively. The suggested deformation mechanism that produces these surface corrugations in the hybrid fibres is illustrated in Figure 3c . Figure 3: Structural changes of hybrid fibres during tensile tests. ( a , b ) SEM images showing the surfaces of hybrid fibres before stretching ( a ) and after fracture ( b ). The arrows of ( a ) and ( b ) indicate the fibre axis. Scale bar equals 1 μm, and the inset scale bar in ( b ) equals 200 nm. ( c ) Schematic illustrations showing structural changes of hybrid fibres generated during tensile tests. Black rectangles, black lines and blue curved lines are RGOFs, SWNTs and PVA chains, respectively. Full size image Carbon nanomaterials and polymer chain alignment in fibres Our strategy for producing super-tough PVA composite fibres was to introduce well-aligned SWNT/RGOF structures that retain a controlled degree of oxidation and a wrinkled topography for the RGOF. Retention of wrinkling results in a highly dispersed state for the RGOF in the polymer matrix [20] , thereby maximizing the fraction of the surface area (up to 2,675 m 2 g −1 ) [21] available for mechanical reinforcement and toughening [11] . Furthermore, we wanted to keep the PVA matrix in a moderately oriented state, so that a large degree of matrix elongation was available during tensile loading for absorbing energy and thereby contributing to toughness. Polarized Raman spectroscopy and X-ray diffraction were used to characterize the degree of alignment of SWNTs and RGOFs in the PVA fibres ( Fig. 4 ). Raman spectra of fibres were collected using a LabRam HR (Jobin-Yvon, France) spectrometer equipped with a confocal microscope that deployed a 514.5-nm Ar-ion laser. The intensity ratio of the Raman G band for light polarized in the direction of fibre axis (G || ) to that for transverse direction polarization is very sensitive to the orientation of CNTs with respect to the fibre axis [22] . A high intensity ratio has been reported for CNT/PVA fibres subjected to postspinning stretch at room temperature [23] . Unlike for these studies, we found that the similarly high-intensity ratios could be achieved for as-spun fibres without the need for a subsequent drawing process ( Fig. 4a ). Strikingly, the intensity ratio increased with increasing RGOF fraction in the hybrid fibre, reaching a maximum for 1:1 RGOF to SWNT loading ( Fig. 4a ), indicating that this ratio of nanocarbons provided the highest degree of alignment during spinning. Further structural characterization of hybrid fibres and polymer-free RGOF fibres, demonstrating the wrinkled nature of the RGOF by using the ratio of intensities of the D peak to G peak (I D /I G ) in the Raman spectra, is shown in Supplementary Figure S2 . The details are described in the 'Methods' section. 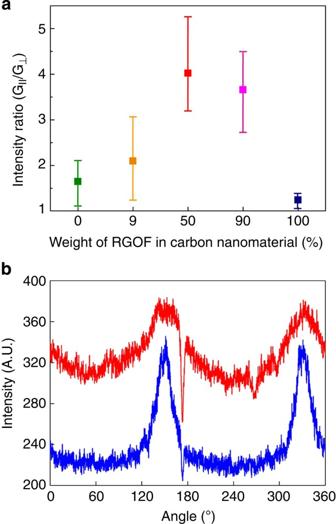Figure 4: Alignment of carbon nanomaterials and polymer chains in polymer composite fibres. (a) Raman intensity ratio for polarization parallel and perpendicular to the fibre axis as a function of wt.% of RGOF in the carbon nanomaterial. (b) Diffraction intensities atQ=1.4 Å−1(a scattering wave vector corresponding to the diffraction from PVA chains) versus fibre orientation angle for hybrid fibres containing equal wt.% SWNTs and RGOFs before (red line) and after (blue line) tensile tests. Error bars inarepresent the minimum and maximum values obtained from five independent experiments. Figure 4: Alignment of carbon nanomaterials and polymer chains in polymer composite fibres. ( a ) Raman intensity ratio for polarization parallel and perpendicular to the fibre axis as a function of wt.% of RGOF in the carbon nanomaterial. ( b ) Diffraction intensities at Q =1.4 Å −1 (a scattering wave vector corresponding to the diffraction from PVA chains) versus fibre orientation angle for hybrid fibres containing equal wt.% SWNTs and RGOFs before (red line) and after (blue line) tensile tests. Error bars in a represent the minimum and maximum values obtained from five independent experiments. Full size image Figure 4b shows the dependence of X-ray scattering intensity on fibre orientation, before and after tensile tests, for hybrid fibres with 1:1 ratio of RGOF to SWNT. These measurements, showing relatively sharp peaks indicative of chain alignment, are for an X-ray wave vector Q =1.4 Å −1 , which corresponds to scattering from partially oriented PVA chains [6] . Similarly sharp peaks were not observed for unstretched RGOF/PVA and SWNT/PVA fibres. Assuming a Gaussian distribution for chain orientation, the half-widths at half-maximum of the peaks for undrawn and drawn hybrid fibres were ±22.2° and ±11.1°, respectively. The decreasing peak width indicates that increased alignment of the PVA chains along the fibre axis is produced by high-fibre stretch during tensile testing. The extent of polymer chain alignment achieved in the undrawn hybrid fibres, as measured by peak half-width, is similar to that previously reported for super-tough CNT/PVA fibres made by cold drawing after spinning (±27°), but significantly smaller than for hot-drawn CNT/PVA fibres (±4.3°) that were considerably less tough [6] . The PVA matrix in our as-spun hybrid fibres is partially aligned, as shown in Figure 4b , and has the capacity for further matrix elongation and alignment during tensile stretch. Fibre morphology and shape setting Evaluation of the fibre fracture surface further reveals the degree of orientation for the network of carbon nanoparticles. Poorly oriented nanoparticles were observed on the fracture surfaces of the RGOF/PVA and SWNT/PVA fibres ( Fig. 5 ). These structures are similar to previously produced undrawn CNT/PVA fibres with a mesh-like structure consisting of unaligned and entangled CNT bundles [7] . The high degree of order formed in the 1:1 hybrid fibres, as indicated by Raman measurements, is absent in these fibres, which are formed by using SDBS dispersion of solely RGOF, due to the inability to form an interconnected network during the spinning and coagulation phase of fibre formation. 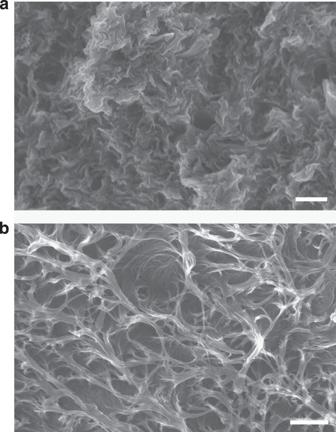Figure 5: Fracture morphology of polymer composite fibres. SEM images of the fracture surfaces of (a) RGOF/PVA and (b) SWNT/PVA fibres. Scale bar equals 500 nm. Figure 5: Fracture morphology of polymer composite fibres. SEM images of the fracture surfaces of ( a ) RGOF/PVA and ( b ) SWNT/PVA fibres. Scale bar equals 500 nm. Full size image SEM of the fracture surface of the as-spun hybrid fibre with 1:1 ratio of RGOF to CNT supports the Raman results by revealing a high degree of SWNT alignment in the fibre direction ( Fig. 6a ). Higher magnification images also showed that the RGOFs were favourably oriented in the fibre direction with SWNT bundles attached to the RGOF edges and surfaces ( Fig. 6b ). Polymer-free hybrid fibres prepared here by spinning into aqueous HCl had a distinct layered structure consisting of wrinkled RGOFs and associated SWNTs ( Fig. 6c ), which is similar to that observed for sheets fabricated by vacuum filtration of dispersions of GOFs [24] . 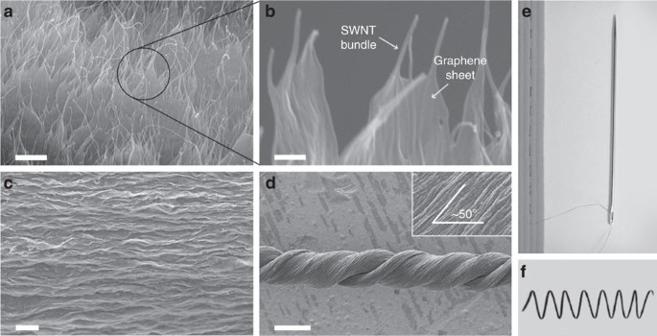Figure 6: Images of fibre structure and a fibre-derived spring. (a) SEM image of a fracture surface showing well-oriented RGOFs and SWNTs in a 1:1 RGOF/SWNT wet-spun hybrid fibre. Scale bar equals 500 nm. (b) Magnified image of the above fracture surface. The scale bar equals 100 nm. (c) SEM image of the layered structure on the surface of a 1:1 hybrid fibre wet spun using a polymer-free coagulation bath. The scale bar equals 1 μm. (d) A 1:1 hybrid PVA composite fibre that has been twisted by using an electric motor. The inset shows the twist angle. The scale bar equals 50 μm. The insert is an SEM image showing the orientation angle of the nanotubes with respect to the fibre axis. (e) Photograph showing a hybrid fibre sewn into a rubber band and an attached 3.5-cm long needle. (f) A spring-shaped hybrid fibre that was set by annealing at 150 °C (spring length: ~6.5 mm, spring diameter: ~1.2 mm and fibre diameter: ~50 μm). Figure 6: Images of fibre structure and a fibre-derived spring. ( a ) SEM image of a fracture surface showing well-oriented RGOFs and SWNTs in a 1:1 RGOF/SWNT wet-spun hybrid fibre. Scale bar equals 500 nm. ( b ) Magnified image of the above fracture surface. The scale bar equals 100 nm. ( c ) SEM image of the layered structure on the surface of a 1:1 hybrid fibre wet spun using a polymer-free coagulation bath. The scale bar equals 1 μm. ( d ) A 1:1 hybrid PVA composite fibre that has been twisted by using an electric motor. The inset shows the twist angle. The scale bar equals 50 μm. The insert is an SEM image showing the orientation angle of the nanotubes with respect to the fibre axis. ( e ) Photograph showing a hybrid fibre sewn into a rubber band and an attached 3.5-cm long needle. ( f ) A spring-shaped hybrid fibre that was set by annealing at 150 °C (spring length: ~6.5 mm, spring diameter: ~1.2 mm and fibre diameter: ~50 μm). Full size image Hybrid fibres with 1:1 ratio of RGOF to SWNT were robust and easily handled. The hybrid fibres could be severely twisted using an electric motor without breaking. The deformation induced by twisting was retained in the fibres to a helix angle of ~50° ( Fig. 6d ). This behaviour shows that the hybrid fibres had both flexibility and toughness. Additionally, they were sufficiently robust to be sewn into rubber bands, as well as cloth ( Fig. 6e ). Those sewn into a rubber band could be reversibly stretched to an elongation of up to 20%. Figure 6f shows shape-controllability and spring properties of the hybrid fibres. The hybrid fibre was coiled on a 1.2-mm diameter stainless steel tube, and then annealed at 150 °C for 1 h to set the helical spring shape. The resulting hybrid fibre spring had a spring constant of ~41 N m −1 ( Supplementary Fig. S3 ) and showed reversible behaviour after both complete compression and 100% elongation. This spring constant was 400 times higher than for springs made from multi-walled CNT yarns that were directly fabricated from CNT forests [25] . Taking account for different geometries, the higher hybrid spring constant suggests ~60 times higher shear modulus than for these previously described neat CNT yarns [25] . What is the origin of this extraordinary toughening that occurs when equal weight fractions of RGOF and CNT are used in the PVA fibres? The stress–strain curves show that high toughness derives from the combination of high elongation-to-break and relatively high-yield strength. High-fibre ductility results from extensive plastic deformation of the PVA matrix during tensile loading, which is permitted because the PVA is not fully aligned during spinning. Characterization of hybrid fibre morphology indicates development of mutually self-aligned CNTs and RGOFs in a partially aligned PVA matrix for the as-spun fibres. As the PVA chains were only partially aligned during solution spinning, further extensive elongation was possible during tensile loading of the fibres. High ductility is also only possible if the reinforcing carbon nanoparticles (CNTs and RGOFs) do not prematurely fail, and this characteristic results from the covalent structures of these nanoparticles. Fibre toughnesses were seen to closely match the extent of carbon nanoparticle alignment, which was found to depend upon RGOF:SWNT ratio. Finally, the wrinkled nature of the RGOF ( Fig. 1d ; Supplementary Fig. S4 ) also ensures that these particles remain well dispersed and interact strongly with the PVA matrix, thereby enhancing modulus and yield strength. Our explanations for the high toughness of the hybrid fibres rely on previous studies of strengthening and toughening in polymer nano-composites, which emphasize the importance of such toughening mechanisms as viscous energy absorption and crack deflection. High-draw ratios were possible in fibres with optimized RGOF:SWNT ratio, as the aligned RGOFs and SWNTs effectively deflect cracks and prevent premature failure, and the partial misalignment of PVA enables energy dissipation. Faber and Evans [26] theoretically demonstrated that platelet-shaped second-phase particles can effectively enhance toughness by deflecting an advancing crack, thereby increasing crack area and reducing stress intensity at the crack tip. Effective crack deflection relies on the platelet particles oriented roughly perpendicular to the crack growth direction, a high-volume fraction of well-dispersed particles and the particles having high-aspect ratio. Raifee et al . [12] suggested that the Faber and Evans [26] model could explain why they observed significantly higher toughness in graphene/epoxy composites in comparison with CNT-epoxies at the same volume fraction of filler. Similar observations have been made for glassy polymers reinforced with small amounts of exfoliated clay particles [27] . Additional toughening mechanisms reported to be operating in the graphene-based composites are related to energy dissipation through viscous sliding or slip between sheets. Wang et al . [13] describe that extensive hydrogen bonding between GOFs and PVA molecules restricts slippage of GOFs and thereby, reduces elongation at break and toughness. A similar reduction in toughness was noted for chemically cross-linked graphene-oxide sheets as a result of reduced sliding of the GOFs [28] . For their tough RGOF/PVA fibres, Wang et al . [13] reported that partial reduction of the GOF allowed some graphene re-stacking that facilitated slip, which resulted in higher elongations and toughness. It was also shown that more extensive reduction of GOF favoured the formation of graphene clusters that were thought to hinder polymer matrix elongation and therefore, again produce reduced toughness. Other reports have also implicated the wrinkled state of graphene as a factor in improving the mechanical properties of graphene-based composites. Unlike for CNTs, the mechanical interaction of RGOF with the surrounding matrix can be enhanced by creating a wrinkled texture of individual graphene platelets that helps to boost interfacial load transfer [11] , [12] . The wrinkled nature of RGOFs arises from the small buckling threshold [29] , [30] and oxygen substitution [31] . Yang et al . [32] describe a 'slide and click' type of deformation in closely packed corrugated RGOF sheets. These studies suggest that the degree of graphene oxidation can have a significant effect on composite toughness. Nanoparticles that interact well with the surrounding matrix can allow for greater matrix extensions and energy dissipation, and facilitate higher toughness. In summary, synergistic toughness enhancement arises for the optimal combination of SWNTs and RGOFs, because the resulting nanoparticle self-alignment and interference with RGOF stacking provide strong interaction with the PVA matrix, enhance crack deflection, and promote plastic deformation of the stretched PVA ( Supplementary Fig. S5 ). Surprisingly, the optimal nanostructure for toughening formed spontaneously during solution spinning of 1:1 dispersions of RGOFs and SWNTs, but was greatly reduced for other ratios of carbon nanoparticles. The results show that this optimal ratio of SWNT and RGOF leads to a high degree of self-alignment during wet spinning ( Fig. 4a ). Partial alignment of the SDS-dispersed CNTs during injection into a PVA solution has been previously ascribed to the shear-flow-induced orientation of the rigid-rod like CNTs [14] . The orientation was stabilized by aggregation of the CNTs during spinning into the PVA solution. SDS is known to be a good dispersing agent for CNTs, because of the strong adsorption of the hydrophobic SDS tail on the CNT surface. As for other colloidal systems, the charged head of the SDS molecule provides electrostatic repulsion that counteracts the natural tendency for aggregation of CNTs due to the van der Waals interactions [33] . Injection of the SDS-stabilized CNTs into a PVA solution causes some of the adsorbed SDS molecules to be replaced through competition by the amphiphilic PVA chains [14] . The result is a decrease in the surface charge on the CNTs and corresponding reduction in the electrostatic repulsion, thereby facilitating coagulation. RGOFs are stabilized and coagulated in the same manner by SDBS and PVA, respectively. In addition, strong interactions that form between CNTs and RGOFs establish an interconnected network when the two nanoparticles are present in the correct proportions. The network is readily oriented during the fibre spinning and stabilized by the coagulation process. The RGOF may act to bind multiple SWNTs and facilitate their alignment in the shear flow. With an incorrect ratio of RGOFs to CNTs, it appears that the interconnected network cannot be formed and the CNT/RGOF alignment is reduced. SEM of the spun fibre ( Fig. 1b ) and transmission electron microscopy of the diluted and dried dispersion ( Fig. 7a ) support this model by indicating that the RGOFs and SWNTs are closely associated. As the RGOFs used in our work are known to contain functional groups such as –COOH [31] , the oxidation of RGOFs was evaluated using X-ray photoelectron spectroscopy ( Supplementary Fig. S6 ). Oxygen-containing groups and aromatic regions with unoxidized benzene rings in RGOFs can be effective for improving dispersion of RGOFs in water and making hybrid nanostructures through π–π interactions with CNTs, respectively. It has been previously reported that strong non-covalent interaction occurs between exfoliated GOFs and SWNTs [34] . Well-dispersed, 20–100nm long SWNTs self-align on graphite surfaces, as shown by scanning tunnelling microscopy by Yanagi et al . [35] Moreover, hydrogen bonding occurs at pH=7 between hydrophilic sulfonate groups (SO 3 − ) on SDBS that is associated with the SWNTs and functional groups like –COOH on RGOFs ( Fig. 7b ) [36] . This interaction can account for the apparent preferential interaction of the SWNTs with the edges or surfaces of the RGOFs. Thereby, RGOF/SWNT hybrids are obtained in a highly dispersed state in water during solution preparation. The atomic percent of oxygen to carbon in RGOFs obtained from X-ray photoelectron spectroscopy was 11.1%. 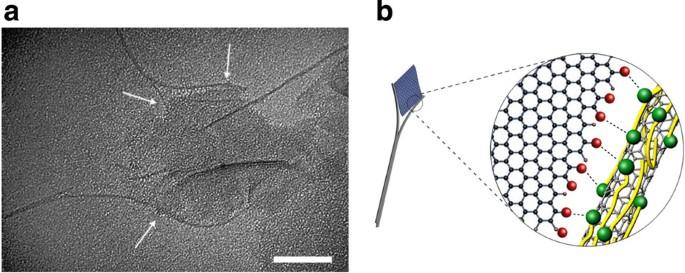Figure 7: Specific interactions between carbon nanomaterials. (a) Transmission electron microscopy image showing the binding of SWNTs with RGOFs. The arrows indicate SWNT bundles. The scale bar equals 100 nm. (b) Schematic diagram showing hydrogen bonding interactions between COOH (red spheres) of RGOFs and SO3−(green spheres) of SDBS (yellow lines) attached to SWNTs. Figure 7: Specific interactions between carbon nanomaterials. ( a ) Transmission electron microscopy image showing the binding of SWNTs with RGOFs. The arrows indicate SWNT bundles. The scale bar equals 100 nm. ( b ) Schematic diagram showing hydrogen bonding interactions between COOH (red spheres) of RGOFs and SO 3 − (green spheres) of SDBS (yellow lines) attached to SWNTs. Full size image In conclusion, we have developed methods for the fabrication of tough composite fibres through the hybridization of wrinkled RGOFs and SWNTs. To our knowledge, the toughness of the hybrid fibres prepared using a 1:1 ratio of RGOF to SWNT exceeds that of any material yet reported, including spider silk and Kevlar. Our fibre preparation method does not require postspinning draw to produce orientation, as mutual self-alignment of RGOFs and SWNTs occurs during spinning when these nanoparticles are present in the correct proportions. The use of RGOFs as a partial substitute for CNTs reduces fibre cost [11] , and facile solution processing can enable upscaled-fibre production. Materials RGOFs, which were stably dispersed in dimethylformamide (DMF) with a concentration of 0.47–0.5 g ml −1 , were used for fibre fabrication. Carbon SWNT (average diameter: 1.3–1.5 nm) powders (ASP-100F) with an average bundle thickness of ~20 nm were purchased from Hanwha Nanotech (South Korea). This SWNT powder has a purity of about 60–70 wt.% (90 vol.%) and contains approximately 10 wt.% of catalyst metal and 20 wt.% of graphitic impurities. The SDBS, methanol and PVA (M w ≈146,000–186,000; hydrolysis ≈99%) were purchased from Sigma-Aldrich and used as received. Preparation of chemically reduced graphene oxide flake RGOF was produced in multi-gram quantities by reduction of an aqueous dispersion of graphene oxide using excess quantities of hydrazine at 95 °C for 2 h [37] . This reduction reaction results in agglomeration of the RGOFs from the aqueous dispersion. These agglomerated RGOF particles were acidified using dilute sulphuric acid to <pH 2 with vigorous stirring and transferred to a sintered glass filter funnel. The agglomerates were washed in the funnel with copious amount of Milli-Q water until the pH of the washing solution was ~7. The filtrand was dried at 70 °C for 48 h under vacuum to give the solid RGOF. This RGOF dry powder was used to prepare a 0.5 mg ml −1 dispersion of RGOF in DMF using ultrasonication under inert atmosphere. The particles of RGOFs were estimated using a Zetasizer, to have an average effective diameter of ~400 nm. This particle size in the dispersion and the zeta potential of the dispersion were stable for several months ( Supplementary Fig. S7 ). Preparation of fibres Aqueous dispersions of RGOF and SWNT were used for fibre spinning. To convert the RGOF/DMF dispersion to an RGOF/water dispersion, the RGOF was collected by centrifugation and the DMF supernatant was removed. The DMF was replaced by an equal volume of water, and then the mixture was ultrasonicated. This process was repeated over three times to ensure that the DMF was largely removed. Next 0.3 wt.% RGOF was dispersed in water using 1 wt.% SDBS surfactant and ultrasonication. The RGOF/water dispersion was then mixed with a dispersion of 0.3 wt.% SWNT in water that was separately prepared using 1 wt.% SDBS surfactant and ultrasonication for 30 min. The RGOF/SWNT dispersion was slowly injected (at a flow rate of 24 ml h −1 through a 26-gauge syringe needle) into a PVA coagulation bath rotating at 10 r.p.m., and continuous and uniform RGOF/SWNT/PVA hybrid fibres were thereby fabricated. The fibres were thoroughly washed in DI water and dried at room temperature, and then they were soaked in methanol for 12 h to increase the crystallinity of the PVA. The ratio of RGOF to SWNTs in the prepared fibres could be easily controlled by adjusting the ratio of the nanoparticles used for the spinning solution. SWNT/PVA and RGOF/PVA fibres were fabricated by the same method, using a 0.3 wt.% SWNT/water solution with 1 wt.% SDBS and a 0.3 wt.% RGOF/water solution with 1 wt.% SDBS, respectively. Characterization Mechanical properties were measured using a thermomechanical analyser (Seiko Exstar 6000, Japan) at a loading rate of 10 mN min −1 . Volumetric fibre toughness (derived by integrating stress–strain curves) was converted to gravimetric fibre toughness by using a fibre density of 2.0 g cm −3 for all PVA composite fibres that contain about 30 wt.% carbon. This approach is consistent with direct measurements that yield a density of ~2.1 g cm −3 for the RGOF/SWNT/PVA hybrid fibres and ~1.9 g cm −3 for the SWNT/PVA fibres. Such densities are higher than would be expected if these fibres did not contain inorganic impurities, such as residual metal catalyst. As high-density, low-volume fraction impurities are unlikely to enhance toughness, the toughness values reported here are likely lower than could be obtained for impurity-free fibres. Diffraction intensities from fibres were measured using a wide-angle X-ray scattering apparatus with a general area diffraction detector (Hi-Star) using incident Cu Kα X-ray radiation. A helium-beam path was used to prevent air scattering. For the transmission electron microscopy (Philips, Model CN30, USA), a small amount of the RGOF/CNT dispersion was further diluted by the addition of water, and a small droplet was dried onto a carbon-film-coated grid. The ratio of D peak to G peak Raman intensities (I D /I G ) in the Raman spectra was ~0.1 for the hybrid fibre, ~0.01 for the CNT/PVA fibre and ~1.3 for the RGOF/PVA fibre, when using 514-nm excitation ( Supplementary Fig. S2a ). We similarly used this Raman ratio at the same excitation wavelength to investigate the degree of wrinkling in hybrid fibres before and after either the acid or thermal treatments to remove PVA. RGOF-based fibres show the defect-induced D band (at ~1,355 cm −1 ), the G band (at ~1,594 cm −1 ), which is related to in-plane vibration of sp 2 carbons, and the two-dimensional peak (at ~2,695 cm −1 ), which is the second order of the D band. The ratio of D to G band intensities (I D /I G ) is related to the size of the sp 2 domains [38] ( Supplementary Fig. S2b ). I D /I G values for pristine RGOF/PVA fibre and polymer-free RGOF fibres were 1.30, 1.26 (acid-treated RGOF fibre) and 0.98 (thermal-treated RGOF fibre), respectively. The decrease of I D /I G resulting from thermal treatment (annealing at 600 °C for 1 h) suggests a possible increase in the average size of the sp 2 domains [31] . Tuinstra and Koenig [39] have noted that I D /I G varies inversely with the crystallite size ( L a ) in graphite: L a (nm)=2.4×10 −10 × λ 4 (I D /I G ) −1 , where λ is the Raman excitation wavelength. Using this relationship, the crystallite sizes (graphitic domain size) of a pristine RGOF/PVA fibre, an acid-treated RGOF fibre and a thermal-treated RGOF fibre were 13.0, 13.3 and 17.1 nm, respectively ( Supplementary Fig. S2c ). This means that acid treatment to remove PVA may generate smaller dewrinkling or unfolding (~2%) of the RGOFs in a fibre than does thermal annealing at 600 °C (~32% dewrinkling or unfolding). However, RGOF fibres that are thermally treated to remove the PVA still have highly wrinkled structures, as shown in the SEM image of Supplementary Figure S4 . The particle size and zeta potential of RGOFs were determined using a Malvern Zetasizer Nano series instrument and a special dip cell kit from this company for non-aqueous samples. The particle size is reported as the equivalent spherical diameter, and only approximately describes the actual dimensions of the quasi two-dimensional RGOF particles. The observed particle size and zeta potential were stable for several months. How to cite this article: Shin, M. K. et al . Synergistic toughening of composite fibres by self-alignment of reduced graphene oxide and carbon nanotubes. Nat. Commun. 3:650 doi: 10.1038/ncomms1661 (2012).